Ordered three-dimensional interconnected nanoarchitectures in anodic porous alumina Three-dimensional (3D) nanostructures combine properties of nanoscale materials with the advantages of being macro-sized pieces when the time comes to manipulate, measure their properties or make a device. However, the amount of compounds with the ability to self-organize in ordered 3D nanostructures is limited. Therefore, template-based fabrication strategies become the key approach towards 3D nanostructures. Here we report the simple fabrication of a template based on anodic aluminium oxide, having a well-defined, ordered, tunable, homogeneous 3D nanotubular network in the sub 100-nm range. The 3D templates are then employed to achieve 3D, ordered nanowire networks in Bi 2 Te 3 and polystyrene. Finally, we demonstrate the photonic crystal behaviour of both the template and the polystyrene 3D nanostructure. Our approach may establish the foundations for future high-throughput, cheap, photonic materials and devices made of simple commodity plastics, metals and semiconductors. Applications of nanomaterials would be undoubtedly ubiquitous, including areas from everyday life to the most advanced science, as they often present new or enhanced properties ascribed to their low dimensionality [1] . However, the practical employment of these nano-sized components into a macroscale device, which must be manufactured in a factory, manipulated by an operator and used in a macroscale world, is frequently hard to carry out. Therefore, the development of high-throughput nanotechnologies for real-life applications has been hitherto relatively slow. A promising strategy towards this goal is to integrate the nano-sized components into a large, hierarchical structure up to the macroscale. Such a material would behave according to the properties of its individual nanocomponents—thus, low-dimensionality effects are expected—while being a macroscale-size piece and, hence, easy to be manipulated and used. Three-dimensional (3D) nanowire-like networks, having a hierarchical architecture comprised of orderly interconnected nanowires, are a good example of these kinds of materials. In fact, they are demonstrating enhanced properties for many applications, as sensors [2] , [3] , electrochromic devices [4] , [5] , solar cells [6] , [7] , energy storage [8] , [9] , [10] , scaffolds with special mechanical properties [11] , optical elements [12] , [13] and for electrocatalysis [14] . Hence, there exists a pressing need for 3D nanofabricated structures. Nevertheless, despite the well-recognized potential of these kinds of 3D nanostructures, their use has been hitherto scarce owing to the lack of scalable methods to synthesize/process functional materials of the desired characteristics. For example, the macroscopic extension of 3D periodic nanostructures restricts their fabrication approaches to those compatible with an affordable large-area production. Therefore, bottom-up fabrication strategies, which exploit the self-organization of building blocks, turn out to be the most appropriate approaches. Unfortunately, the amount of compounds that have the ability to self-organize in 3D periodic structures is limited [15] , which avoids the direct employment of this approach for most of the functional materials. A promising alternative method for periodic 3D nanowire-like networks composed of those materials that do not present self-organizing capabilities is the use of appropriate templates. These templates must present, on one hand, the inverse morphology of the target nanostructure, that is, a 3D nanotubular network, and, on the other hand, a macroscopic extension. Thus, currently, the main challenge in the fabrication of 3D periodic nanowire-like networks is the development of versatile templates with periodic (ordered) 3D nanotubular networks. Gyroid-forming block copolymers—with sacrificial continuous domains—have recently demonstrated to be efficient platforms to integrate 3D templates for the preparation of 3D nanostructures in Au (ref. 12 ), NiO (ref. 5 ), V 2 O 5 (ref. 10 ), TiO 2 (ref. 16 ) by electrodeposition or sol–gel reactions. Likewise, 3D Pt nanowire networks have been also produced by electrodeposition within a track-etched polymer 3D membrane [14] . Both kinds of polymer templates have shown their suitability for the growth of inorganic compounds by non-aggressive, wet-chemical approaches. However, growth methods yielding inorganic materials with the best compositional and crystallographic features, which will eventually present the best properties, such as, atomic layer deposition, molecular beam epitaxy, chemical vapour deposition and the like, commonly imply/need aggressive reaction conditions namely, high temperatures, high vacuum or presence of highly reactive species, which are hardly supported by polymer templates. Thus, block copolymer templates and most of the track-etched templates are not compatible with many of these growth techniques, which avoids the nanostructuration of an important set of inorganic materials by this approach. Note that gyroid 3D nanotubular network structures are frequently conformed in polymers as polystyrene (PS), poly(ethyleneoxide) and so on, which present a working temperature <100 °C. Furthermore, the low surface energy of polymeric templates ( γ polymers <50 mN m −1 ) might hinder the infiltration of other low-surface-energy liquid compounds, such as most of the organic liquids—polymer solutions and melts, liquid crystals and the like—into the tubular space. This would prevent making 3D nanowire-like networks composed of many functional organic materials. In this work, we present the fabrication of a well-defined, controllable, homogeneous periodic 3D nanotubular network over cm 2 areas in anodic aluminium oxide (AAO), with tens of micron thickness and high aspect-ratio. The produced template is composed of alumina, so it is mechanically, chemically and thermally stable and possesses high-surface-energy hydroxilated pore walls, which may promote the infiltration of low-surface-energy fluids. The 3D AAO presented here consists of a hexagonal array of longitudinal nanopores, which are perpendicularly interconnected through transversal nanochannels. Thus, it constitutes a perfectly ordered 3D nanoarchitecture in porous alumina, in contrast to other analogous materials previously reported [17] , [18] , [19] . Such transversal nanochannels thus form networks confined into planes parallel to the alumina surface. The used fabrication approach is inspired by the ‘potentiostatic pulsed anodization’ developed by Lee et al. [20] , [21] , in which mild anodization (MA) and hard anodization (HA) steps are alternated [20] , [22] , [23] . However, in our approach, during HA steps the current is limited to a defined value. Then, we take advantage of the higher etching rates of the aluminium oxide grown under HA [20] to attack selectively those regions, in such a way that longitudinal nanopores become interconnected with their first neighbours through transversal nanochannels. The amount and position of the pore-interconnecting junctions of the tubular network can be precisely adjusted just by selecting the amount and the length of the MA steps. Owing to the adjustable, dense and ordered 3D nanoporous structure, the 3D AAOs presented here can be used as templates for the fabrication of 3D periodic nanowire-like networks in a wide variety of materials with applications in thermoelectricity [24] , catalysis [25] , filtration [26] , energy storage [10] and photonics [2] to name some. Moreover, we show here our results on the fabrication of 3D nanowire-like periodic nanostructures using 3D AAO templates. Thereby, 3D nanowire-like periodic nanostructures made of PS, by in situ polymerization, and Bi 2 Te 3 , by electrodeposition, were fabricated [27] , [28] , [29] to demonstrate the suitability of our templates to fabricate nanowire networks for both organic and inorganic materials using different growth techniques. Finally, the one-dimensional (1D) photonic crystal behaviour of both the 3D AAO and a 3D periodic nanowire-like network made of a commodity plastic as PS is demonstrated, which opens up the possibility to produce high-throughput, cheap, photonic materials and devices made of simple commodity plastics. Anodization processes During a typical pulse anodization process, MA and HA constant voltage steps are periodically alternated [20] , [22] , [23] . However, in our approach while constant voltage is applied in MA steps, the current is limited to a defined value during HA steps and thereof the voltage is not kept constant. The material is grown thus at a defined current during HA periods. Then, the obtained AAO is selectively etched. As a consequence, the aluminium oxide grown under HA is partially removed, so that transversal nanochannels are formed, thus establishing the 3D porous network. Since our aim is to achieve a periodic 3D structure, the ordering of the longitudinal pore arrangement must not be disturbed as a consequence of the alternation of HA and MA steps. From a practical point of view, this means that the AAO layers grown under MA conditions and under HA must present the same latticing parameter of the hexagonal pore arrangement ( D int,long ). D int,long is proportional to the applied voltage in both MA and HA regimes, but the proportionality coefficient, ζ , is different in each of them. The D int,long is 65 nm for an AAO grown in MA conditions under a voltage ( V MA ) of 25 V, so that one should carry out the HA pulses at a voltage leading to the same D int,long value. According to Schwrim et al. [30] , the relationship between D int,long and the applied voltage in the potentiostatic HA regime is ζ HA =1.8 nm V −1 . Thus, the applied voltage during the pulses should be 36 V. However, we experimentally observe that when applying pulses of 36 V without limiting the current intensity, we are not able to grow 3D AAO with a homogeneous porous structure, as the high current during pulses induced severe damages in the structure—probably due to heating effects. We managed to solve this problem by limiting the intensity during the pulses ( I HA ) to 55 mA (that is, a current density, j , of 27.5 mA cm −2 ). Moreover, the current limitation assures that the kinetics of the reaction during the pulses is almost independent of reaction time, so that the same AAO thickness grows in each pulse ( Fig. 1a ). Note that the amount of material grown is directly proportional to j during anodization [31] , [32] . In contrast, when one directly pulses between constant voltage during MA steps ( V MA ) and constant voltage during HA pulses, the current at the HA pulses ( I HA ) decreases with time [20] as the pore become longer and, thus, the growth of the AAO turns to be dependent of the anodization time, which leads to a non-homogeneous network structure in the AAO template (see Supplementary Fig. 1 and Supplementary Note 1 ). This issue is avoided by our procedure. Due to the limitation of current to 55 mA, the maximum voltage ( V HA ) reached during the pulses is 31–31.5 V (see Fig. 1b ), so we fix the nominal applied voltage for the pulses ( V HA,N ) to 32 V. The length of the pulse ( t HA ) is established in 2 s, as we observe that the AAO layer grown during such a pulse is appropriate to afterwards develop transversal nanochannels of the desired dimensions (a few tens of nanometres). Furthermore, we observe that even if we do not anodize exactly at a V HA,N giving rise to a D int ,long of 65 nm, a 2-s pulse is too short a time for the system to lose its order—as shown in Supplementary Fig. 2 ; Supplementary Note 2 . Hence, a 3D AAO is achieved with a highly regular morphology. On the other hand, the length of the MA ( t MA ) steps is varied to tailor the distance between transversal nanochannels, as shown below. 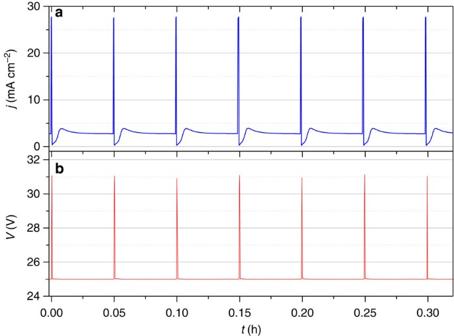Figure 1: Pulse anodization. Current density–time (a) and voltage–time (b) transients during pulse anodization. The anodization process consists of a periodic alternation of mild anodization (MA) steps followed by hard anodization (HA) steps. The maximum current density is fixed at 55 mA. Figure 1: Pulse anodization. Current density–time ( a ) and voltage–time ( b ) transients during pulse anodization. The anodization process consists of a periodic alternation of mild anodization (MA) steps followed by hard anodization (HA) steps. The maximum current density is fixed at 55 mA. 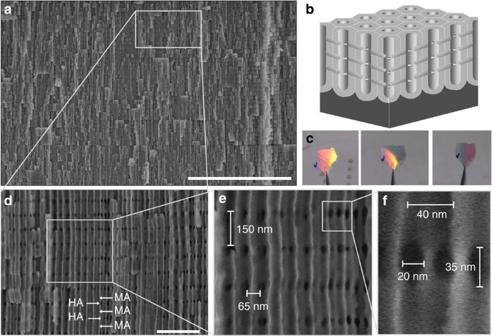Figure 2: 3D anodic alumina template. (a) Representative cross-section SEM image of the 3D AAO template fabricated by pulse anodization (VMA=25 V,tMA=100 s;VHA,N=32 V,tHA=2 s) and subsequent partial chemical etching of the HA regions with H3PO45 wt%, at 30 °C, for 18 min. The sample has being broken to see the cross-section more clearly. Scale bar, 5 μm. (b) Schematic cartoon of the interconnected nanochannel network structure of the 3D AAO templates. (c) Optical photographs of a 3D AAO acquired from different viewing angles (the sample is suspended with tweezers). The arrow indicates the rotation direction. (d) Cross-section micrograph of a 3D AAO template, in which the nanostructure of the template can be appreciated. Scale bar, 500 nm. (e) Enlarged view of the area marked indwith a rectangle, in which both the longitudinal pores (in the vertical direction) and the transversal pores (in the horizontal and in the out-of-plane direction of the image) can be distinguished. The distance between longitudinal nanopores (Dint,long) is 65 nm, while the separation of the planes containing the transversal nanopores (Dint,trans) is 150 nm for this specific 3D AAO. (f) Detailed view of the nanochannel structure from which the dimensions of different nanopores can be measured. The diameter of longitudinal nanopores is 40 nm. The section of the transversal nanochannels is rather ellipsoid, presenting a short diameter of 20 nm and a large diameter of ~35 nm. Full size image The 3D AAO template Figure 2a shows a representative scanning electron microscope (SEM) image of a longitudinal fracture surface of the 3D AAO template fabricated by pulse anodization ( V MA =25 V, t MA =100 s; V HA,N =32 V, t HA =2 s) and subsequent partial chemical etching of the HA regions with H 3 PO 4 5 wt%, at 30 °C, for 18 min. Longitudinal pores laid on the vertical direction, while transversal nanochannel layers are arranged along the horizontal and the out-of-plane directions of the image. Thereby, the 3D nanochannel network in the 3D AAO consists of a set of parallel longitudinal nanopores, such as those formed via a constant voltage anodization process in ‘common’ AAO templates, and transversal nanochannels, which interconnect adjacent longitudinal nanopores at some periodic points. The tubular network structure is thus similar to that of the illustration in Fig. 2b . The MA/HA-alternating layer structure of the 3D AAOs induced the appearance of structural colour in the 3D AAO, as both layers have different refracting indexes and are periodically alternated. The 3D AAO thus behaves as a distributed Bragg reflector (DBR) or a 1D photonic crystal, as can be observed in Fig. 2c , in which optical images of the 3D AAO acquired from different viewing angles are shown. The change in colour can be appreciated while rotating the sample. Such an alternating-layered structure can be clearly appreciated in the cross-sectional SEM image in Fig. 2d . Figure 2: 3D anodic alumina template. ( a ) Representative cross-section SEM image of the 3D AAO template fabricated by pulse anodization ( V MA =25 V, t MA =100 s; V HA,N =32 V, t HA =2 s) and subsequent partial chemical etching of the HA regions with H 3 PO 4 5 wt%, at 30 °C, for 18 min. The sample has being broken to see the cross-section more clearly. Scale bar, 5 μm. ( b ) Schematic cartoon of the interconnected nanochannel network structure of the 3D AAO templates. ( c ) Optical photographs of a 3D AAO acquired from different viewing angles (the sample is suspended with tweezers). The arrow indicates the rotation direction. ( d ) Cross-section micrograph of a 3D AAO template, in which the nanostructure of the template can be appreciated. Scale bar, 500 nm. ( e ) Enlarged view of the area marked in d with a rectangle, in which both the longitudinal pores (in the vertical direction) and the transversal pores (in the horizontal and in the out-of-plane direction of the image) can be distinguished. The distance between longitudinal nanopores ( D int,long ) is 65 nm, while the separation of the planes containing the transversal nanopores ( D int,trans ) is 150 nm for this specific 3D AAO. ( f ) Detailed view of the nanochannel structure from which the dimensions of different nanopores can be measured. The diameter of longitudinal nanopores is 40 nm. The section of the transversal nanochannels is rather ellipsoid, presenting a short diameter of 20 nm and a large diameter of ~35 nm. Full size image The dimensions of the structural features of a 3D AAO obtained after 60 MA/HA repetitions ( V MA =25 V, t MA =100 s; V HA,N =32 V, t HA =2 s) and the subsequent etching process in H 3 PO 4 5 wt%, at 30 °C, for 18 min are shown in Fig. 2d–f . The total area of the 3D template is 2. In the direction perpendicular to the template surface, the thickness of the 3D porous structure is ~20 μm (only about 10 μm are shown in Fig. 2a ), but it can be increased through a higher amount of MA/HA repetitions. Hence, the whole 3D porous network has macroscale dimensions. In contrast, the structure of the network is entirely nanoscopic. The distance between longitudinal nanopores ( D int,long ) is 65 nm, while the distance between planes containing the transversal nanopores ( D int,trans ) is 150 nm for this specific 3D AAO example ( Fig. 2e ). Longitudinal nanopores present a diameter of 40 nm due to the pore-widening process (originally, pores that are 25 nm in diameter are obtained), as observed in Fig. 2f . In such micrographs, longitudinal nanopores lay vertically and the transversal nanochannels lay out-of-plane of the image. The diameter of transversal nanochannels depends on the chemical etching process. For the typical etching process indicated above, the section of the transversal nanochannels is rather ellipsoid, presenting a short diameter of 20 nm and a large diameter of ~35 nm ( Fig. 2f ). Although the 3D porous architecture in 3D AAOs is a consequence of the pulsed anodization, only 1D longitudinal nanopores are originally formed due to the anodization process, as can be observed in Fig. 3a . However, the alumina grown under HA conditions is chemically less stable than that grown under MA conditions, as found by Lee et al. [20] Thereby, the chemical etching rate of the alumina grown under HA is significantly higher than of that grown under MA. In this way, when the AAO is attacked with an acid solution, AAO regions formed during the HA pulse are preferentially dissolved. Hence, one may preferentially widen the longitudinal nanopores in the HA regions until each longitudinal pore collapses with the next neighbour, without significantly affecting the longitudinal nanopore regions formed under MA steps, thus creating transversal nanochannels between longitudinal nanopores ( Fig. 3b ). 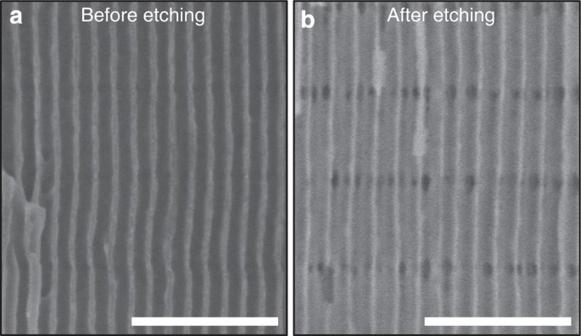Figure 3: Formation of the 3D porous network. Cross-sectional SEM image of a 3D AAO prepared by pulsed anodization before (a) and after (b) the chemical etching process in H3PO4(H3PO45 wt%, at 30 °C, for 18 min). Scale bar, 500 nm. Figure 3: Formation of the 3D porous network. Cross-sectional SEM image of a 3D AAO prepared by pulsed anodization before ( a ) and after ( b ) the chemical etching process in H 3 PO 4 (H 3 PO 4 5 wt%, at 30 °C, for 18 min). Scale bar, 500 nm. Full size image Geometry of the 3D network Longitudinal pores are orderly fashioned due to the fact that both the first anodization and the MA steps of the pulse anodization is carried out in self-ordering conditions (25 V, 0 °C, 0.3 M H 2 SO 4 ) ( Supplementary Fig. 2 ; Supplementary Note 2 ). This hexagonal pore distribution is not disturbed by the HA steps, as can be observed in the Supplementary Fig. 2c . Therefore, longitudinal nanopores are completely parallel along the entire thickness of the template. To assess the geometry of the transversal nanochannel network, we analyse the morphology of an internal MA terrace after the detachment of the upper layers ( Fig. 4a ). A close view of its surface ( Fig. 4b ) reveals that the transversal nanochannels conform a 2D porous network of hexagonal symmetry (see also Supplementary Fig. 3 ; Supplementary Note 2 ). This is obviously a consequence of the hexagonal order of the longitudinal nanopore array. Hence, the nanoporous network of the 3D AAO consists of a hexagonal array of longitudinal nanopores, which are perpendicularly interconnected through the transversal nanochannel network, presenting also hexagonal symmetry (see also ( Supplementary Fig. 4 ). 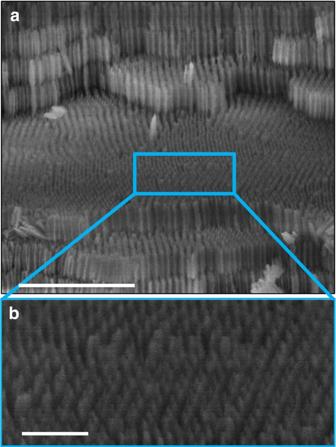Figure 4: Geometry of transversal nanochannels. (a) SEM micrograph of a fracture of a 3D AAO showing a MA terrace after the detachment of the upper layers. Scale ba, 1 μm. And, (b) the transversal nanochannel networks present a hexagonal symmetry as illustrated in the detailed view. Scale bar, 200 nm It can be observed they are well aligned. Figure 4: Geometry of transversal nanochannels. ( a ) SEM micrograph of a fracture of a 3D AAO showing a MA terrace after the detachment of the upper layers. Scale ba, 1 μm. And, ( b ) the transversal nanochannel networks present a hexagonal symmetry as illustrated in the detailed view. Scale bar, 200 nm It can be observed they are well aligned. Full size image We have tried to extract further information about the HA layer by means of ellipsometry ( Supplementary Figs 5 and 6 ), which gives access to its refractive index and thus can be related to morphological parameters such as the porosity of the layer. For that, a sample is fabricated containing a single transversal nanochannel plane sandwiched between two MA layers, and the ellipsometric data were fixed with a five-layer model that took the fundamental parameters (as described in the Supplementary Note 3 ). The obtained porosity for the HA layer accounts to 75%. Tuning geometry of the 3D nanoporous network In contrast to previous attempts to fabricate 3D structures in AAO, the procedure presented in this work allows a precise control over the morphology of the material. In the approach by Lee et al. [17] the spontaneous current oscillations taking place during the HA process in oxalic acid electrolyte induced pore diameter modulations, which can be eventually used to prepare a 3D porous network. Nevertheless, although they showed a well-defined 3D porous structure at a local scale, the achieved porous network lacked structural homogeneity along both the in-plane and the cross-plane directions, due to the fact that the formation of the network is a consequence of self-induced current oscillations, which are difficult, if not infeasible, to be controlled. Therefore, one cannot adjust the period, the shape and the amplitude of the diameter modulations by their approach and, in consequence, neither the morphology of the 3D porous network. Furthermore, the AAO template they obtained presented a thickness distribution over the film. Likewise, in Losic’s [19] , [33] and Wang’s [18] approach, the non-perfect organization of longitudinal pores together with lengthy etching treatments required for interconnecting the longitudinal pores led to severe structural damages in the material. On the contrary, one can precisely adjust the amount and position of the pore-interconnecting junctions of the tubular network through our approach, just by selecting the amount and the length of the MA regions, as it can be observed in Fig. 5 . Moreover, since every single step in the anodization processes is well controlled and homogeneous, we can achieve well-defined 3D porous structures with no structural defects. Thereby, we fabricate 3D AAOs having different distances between transversal nanochannel regions/planes. 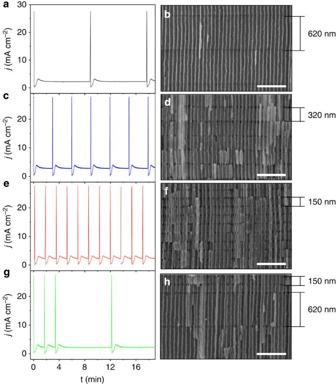Figure 5: Modulation of the distance between transversal nanochannels. I–ttransients of pulsed anodizations in which thetMAhas been varied: (a)tMA=530 s, (c)tMA=180 s, (e)tMA=100 s. (g) TheI–tplot of a pulsed anodization in which two differenttMAhave been applied:tMA, 1=100 s andtMA, 2=530 s. SEM images of the AAOs obtained thereof are shown inb,d,fandh, respectively. The distance between transversal nanochannels are: (b) 620 nm (tMA=530 s), (d) 320 nm (tMA=180 s) and (f) 150 nm (tMA=100 s). When two distincttMAare applied, an AAO with two different separations between transversal nanochannels can be prepared, as evidenced inh. Scale bars, 500 nm. Figure 5b,d,f shows 3D AAOs in which such a distance is tailored to 620 nm ( t MA =530 s, Fig. 5a ), 320 nm ( t MA =180 s, Fig. 5b ) and 150 nm ( t MA =100 s, Fig. 5c ), respectively. Moreover, one can also prepare a single 3D AAO with different distances between transversal nanopores, such as that shown in Fig. 5h . Note that by tailoring the amount and position of the transversal nanopores we modulate the density of integration of the eventual 3D periodic nanowire-like network formed within the 3D AAO, with the subsequent modulation of its properties (optical, mechanical, thermoelectric and so on). Figure 5: Modulation of the distance between transversal nanochannels. I–t transients of pulsed anodizations in which the t MA has been varied: ( a ) t MA =530 s, ( c ) t MA =180 s, ( e ) t MA =100 s. ( g ) The I–t plot of a pulsed anodization in which two different t MA have been applied: t MA, 1 =100 s and t MA, 2 =530 s. SEM images of the AAOs obtained thereof are shown in b , d , f and h , respectively. The distance between transversal nanochannels are: ( b ) 620 nm ( t MA =530 s), ( d ) 320 nm ( t MA =180 s) and ( f ) 150 nm ( t MA =100 s). When two distinct t MA are applied, an AAO with two different separations between transversal nanochannels can be prepared, as evidenced in h . Scale bars, 500 nm. Full size image 3D nanostructures composed of functional materials Finally, we show here our results on the fabrication of 3D nanostructures using the 3D AAO templates. 3D nanowire-like periodic nanostructures made of Bi 2 Te 3 and other polymers such as PS have been fabricated [27] , [28] , [29] to demonstrate the suitability of our templates both to grow 3D organic and inorganic materials. 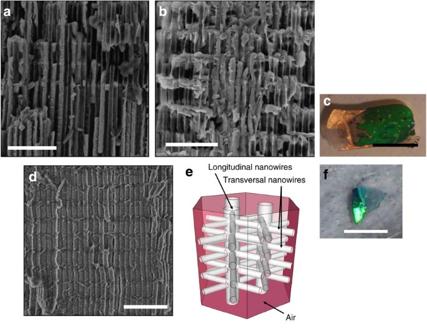Figure 6: 3D Bi2Te3and 3D PS nanostructured materials. (a,b) Cross-sectional SEM micrographs of a three-dimensional periodic nanostructure (3D periodic nanostructures) of the semiconductor Bi2Te3electrodeposited inside a 3D AAO template (VMA=25 V,tMA=180 s,VHA,N=32 V,tHA=2 s). Scale bars, 500 nm. (c) Optical photograph of the template after Bi2Te3filling, the black bar is 1 cm. (d) Cross-sectional SEM micrograph of a three-dimensional periodic nanostructure (3D-periodic nanostructures) of polystyrene (PS) after removal of the 3D AAO (VMA=25 V,tMA=180 s,VHA,N=32 V,tHA=2 s). Scale bars, 500 nm. (e) Sketch of the observed interconnected nanowire array. And (f) optical photograph of the freestanding polystyrene 3D nanowire network after alumina removal, the black bar is 1 cm. Figure 6a,b shows the cross-sectional SEM images of a 3D AAO containing a Bi 2 Te 3 3D periodic nanowire-like network prepared by pulsed electrodeposition [34] . Figure 6c shows an optical photograph of the material, in which the green-coloured area is where the Bi 2 Te 3 was grown and the yellow areas correspond to the gold substrate used as an electrode. The scale bar corresponds to 1 cm in this image. Note the change in colour due to the Bi 2 Te 3 nanowire network as compared with empty 3D AAO ( Fig. 2c ) or the black colour when nanowires are prepared in a conventional AAO template. Figure 6: 3D Bi 2 Te 3 and 3D PS nanostructured materials. ( a , b ) Cross-sectional SEM micrographs of a three-dimensional periodic nanostructure (3D periodic nanostructures) of the semiconductor Bi 2 Te 3 electrodeposited inside a 3D AAO template ( V MA =25 V, t MA =180 s, V HA,N =32 V, t HA =2 s). Scale bars, 500 nm. ( c ) Optical photograph of the template after Bi 2 Te 3 filling, the black bar is 1 cm. ( d ) Cross-sectional SEM micrograph of a three-dimensional periodic nanostructure (3D-periodic nanostructures) of polystyrene (PS) after removal of the 3D AAO ( V MA =25 V, t MA =180 s, V HA,N =32 V, t HA =2 s). Scale bars, 500 nm. ( e ) Sketch of the observed interconnected nanowire array. And ( f ) optical photograph of the freestanding polystyrene 3D nanowire network after alumina removal, the black bar is 1 cm. Full size image Moreover, a 3D nanowire-like network is also fabricated in PS. Figure 6d shows the cross-section of such a material after the removal of the 3D AAO template in NaOH. Thus a freestanding network of nanowires is shown as is represented in Fig. 6e . Note that the greenish colour of Fig. 6f is due exclusively to the nanoarchitecture, since bulk PS is transparent. The scale bar corresponds to 1 cm in this image. This example constitutes a clear demonstration of the efficacy of our template to nanostructure low-surface-energy materials. Other examples of functional polymers infiltrated in 3D AAO templates are shown in Fig. 7 . 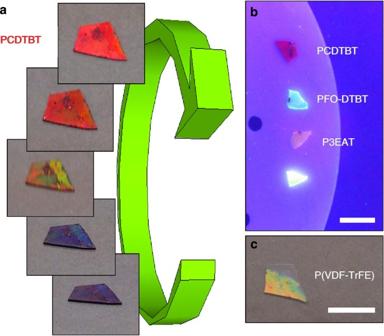Figure 7: 3D AAO-functional polymer composite materials. (a) Optical images of a 3D AAO (VMA=25 V,tMA=180 s,VHA,N=32 V,tHA=2 s) infiltrated with PCDTBT polymer observed from different rotation angles. A video recorded with a cellphone can be found in theSupplementary Movie 1. (b) Photographs of 3D AAO templates infiltrated with different conjugated polymers acquired under dark light. From top: PCDTBT, a copolymer based on fluorene, thiophene and benzothiazole (PFO-DTBT), poly(3-ethyl acetate thiophene-2,5-diyl) (P3EAT) and poly(phenylene vinylene) (PPV). Scale bars, 1 cm. (c) Photographs of a 3D AAO template infiltrated with the ferroelectric polymer poly(vinylidene flouride-co-trifluoroethylene) (PVDF-TrFE). Scale bars, 1 cm. Figure 7a shows a set of photographs (from different viewing angles) of the conjugated polymer poly[[9-(1-octylnonyl)-9H-carbazole-2,7-diyl]-2,5-thiophenediyl-2,1,3-benzothiadiazole-4,7-diyl-2,5-thiophenediyl] (PCDTBT) inside 3D AAO ( V MA =25 V, t MA =180 s, V HA,N =32 V, t HA =2 s). The different colours observed as a function of the eye angle are the direct consequence of the diffraction grating generated by the PCDTBT-filled transversal nanochannels and the alumina layers ( Supplementary Movie 1 , recorded with a cellphone). More examples of light-emitting materials prepared by infiltrating conjugated polymers such as the copolymer based on fluorene, thiophene and benzothiazole, poly(3-ethyl acetate thiophene-2,5-diyl), poly(phenylene vinylene)) into 3D AAOs are presented in Fig. 7b . The photographs are acquired under black light. Finally, composite materials showing complex response—electrical and optical for instance—can be prepared by infiltrating an electroactive polymer—such as the ferroelectric poly(vinylidene flouride-co-trifluoroethylene)—into the 3D AAO ( Fig. 7c ). Figure 7: 3D AAO-functional polymer composite materials. ( a ) Optical images of a 3D AAO ( V MA =25 V, t MA =180 s, V HA,N =32 V, t HA =2 s) infiltrated with PCDTBT polymer observed from different rotation angles. A video recorded with a cellphone can be found in the Supplementary Movie 1 . ( b ) Photographs of 3D AAO templates infiltrated with different conjugated polymers acquired under dark light. From top: PCDTBT, a copolymer based on fluorene, thiophene and benzothiazole (PFO-DTBT), poly(3-ethyl acetate thiophene-2,5-diyl) (P3EAT) and poly(phenylene vinylene) (PPV). Scale bars, 1 cm. ( c ) Photographs of a 3D AAO template infiltrated with the ferroelectric polymer poly(vinylidene flouride-co-trifluoroethylene) (PVDF-TrFE). Scale bars, 1 cm. Full size image Optical properties of the 3D AAO and nanowire networks The optical properties of the 3D AAO were investigated by ultraviolet–visible spectroscopy. The reflectance spectrum obtained from a 3D AAO constructed on a glass substrate is seen in Fig. 8a . The distance between transversal nanochannels was 320 nm in this sample, whereas the number of MA/HA bilayers amounted to 60. Both the reflectance and transmittance spectra (in the Supplementary Fig. 7 ) show a well-defined optical band gap centred at ≈650 nm, as corresponding to a periodicity of ≈320 nm (see the SEM micrograph in Fig. 8b ). Note that an analogous porous alumina having only longitudinal nanopores (named as ‘common AAO’) shows an almost flat reflectance ( Fig. 8c ) and transmittance spectra ( Supplementary Fig. 7 ). Thus, the 3D AAOs enable one to easily fabricate highly tunable DBRs in which both the distance between the alternating layers and the refraction index can be fully modulated. The periodicity can be easily modulated through the length of the MA periods, while the refraction index can be tuned by infiltrating the 3D template with materials having the desired refractive index, such as polymers from solutions (for example, following the approach showed in the Fig. 7 ). Note that this 3D AAO might also serve to fabricate better DBR and anisotropic 3D photonic structures, as its photonic properties will be different in the in-plane and cross-plane directions. But, more interesting are the optical properties of the 3D nanowire networks fabricated from the 3D AAO. We demonstrate here that by employing 3D AAOs, one can easy produce cheap 1D photonic crystals, even made of a ‘simple’ and popular commodity plastic as PS. 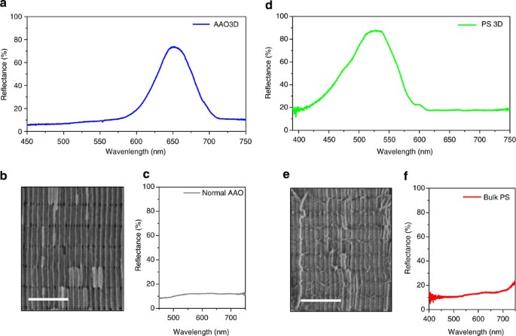Figure 8: Optical properties of 3D nanostructuctures. (a) Reflectance spectrum obtained from the 3D AAO shown inb. (c) Reflectance spectrum of an AAO without transversal nanocannels (named as ‘common AAO’). (d) Reflectance spectra of the PS nanowire network shown ine. (f) Reflectance spectrum of a non-porous PS (named as ‘bulk PS’). Scale bars in SEM micrographs correspond to 500 nm. Figure 8d shows the reflectance spectrum of the PS 3D nanowire network shown in Fig. 8e . Again, an intense reflection band at ≈525 nm can be observed as a consequence of the alternation of layers with different refractive indices. This reflection band at ≈525 nm is responsible for the strong green colour of this PS piece. Note that bulk PS is absolutely colourless. The PS nanowire network was prepared form a 3D AAO having a periodicity of ≈320 nm; however, the band gap in the PS 3D nanostructure is blue-shifted (≈525 nm) probably as a consequence of a shrinkage or relaxation process of the nanostructure after the 3D AAO template removal. Figure 8: Optical properties of 3D nanostructuctures. ( a ) Reflectance spectrum obtained from the 3D AAO shown in b . ( c ) Reflectance spectrum of an AAO without transversal nanocannels (named as ‘common AAO’). ( d ) Reflectance spectra of the PS nanowire network shown in e . ( f ) Reflectance spectrum of a non-porous PS (named as ‘bulk PS’). Scale bars in SEM micrographs correspond to 500 nm. Full size image A nanoporous AAO template has been prepared having a well-defined and homogeneous periodic 3D nanotubular network. The used fabrication approach includes a new type of pulsed anodization process, in which MA and HA pulses are alternated. The voltage here is maintained constant during MA steps, while during HA pulses the current is limited to a fixed value. This current limitation is responsible for the high uniformity of the 3D nanostructure over the macroscopic piece, which yields a real 3D ordered nanostructure. The preferential chemical etching of the aluminium oxide grown under HA regime led then to the formation of transversal nanochannels, which interconnect adjadcent longitudinal nanopores. The 3D AAO thus formed consists of a hexagonal array of longitudinal nanopores, perpendicularly interconnected through transversal nanochannels. 3D nanoporous networks with a thickness >20 μm in the template cross-plane direction are prepared, but size limitation on this matter is not expected. Likewise, the lateral extension of the network prepared is in the order of cm 2 and limitations are neither expected. The number and the distance between planes containing the transversal nanopores can be precisely tailored selecting the amount and the length of the MA steps, which allow the modulation of the pore density of the templates. The distance between longitudinal nanopores is 65 nm. The diameter of longitudinal nanopores is 40 nm, while the section of the transversal nanochannels, which is ellipsoid, presents a short diameter of 20 nm and a large diameter of ~35 nm. 3D AAOs serve as templates for the fabrication of 3D periodic nanowire-like networks in a wide variety of materials with applications in thermoelectricity, catalysis, filtration, energy storage, photonics and the like. Thereby, we show the first attempts to the fabrication of 3D periodic nanowire-like nanostructures made of PS and Bi 2 Te 3 , as well as 3D composite nanostructures comprised of functional polymers. The development of such a versatile, rapid, low-cost, industrially scalable processing route that allows efficient and controlled deposition of materials into structures with complex behaviour and complex geometries—Al pieces having any shape can be anodized—can be expected to impinge on a variety of fields, from information lighting, to sensing, to coating, to biomedicine. Thereby, we have demonstrated the 1D photonic crystal behaviour of both the 3D AAO and a 3D periodic nanowire-like network made of a commodity plastic such as PS. Hence, through these new materials and procedures, we might be presenting here the foundations for future high-throughput, cheap, photonic materials and devices made of simple commodity plastics. Preparation of the 3D AAO templates The 3D-AAO templates were prepared by a two step anodisation method [35] , in which the second step was a pulsed anodisation process. To begin with, ultrapure (99.999%) aluminium foils (Advent Research Materials, England), were cleaned and degreased by sonication in acetone, water, isopropanol and ethanol. Foils were then electropolished in a solution of perchloric acid/ethanol (1/3) under a constant voltage of 20 V for 4 min. After that, the first anodization was achieved for 24 h. A 0.3-M sulphuric acid (Panreac AC Química, Spain) solution was used under a voltage of 25 V and at 0 °C. Then, the first anodic layer was removed by chemical etching in a mixture of phosphoric acid (7 wt%) and chromic oxide (1.8 wt%). A pulsed anodization process was then carried out in the conditions specified along the text. Afterwards, the underlying aluminium substrate was etched with an acidic solution of CuCl 2 at 1 °C and the barrier layer was dissolved using a 10 wt% aqueous H 3 PO 4 solution at 30 °C. Finally, the samples were submerged into a 5 wt% aqueous H 3 PO 4 solution at 30 °C to create the transversal nanochannels. Characterization The morphology study of 3D AAO was performed by SEM (Hitachi SU8000) operating at an accelerating voltage of 2 kV to avoid the deposit of any conducting layer and charging. The microscope had been properly calibrated by the operators from Hitachi Ltd. Also, the accuracy of the measurement was checked in previous works. Ellipsometry measurements were carried out (M2000FI J.A. Woollam Co.) between 350 and 1,640 nm wavelengths and with incidence angles of 50°, 60° and 70°. The samples specifically prepared for ellipsometry measurements are described in the Supplementary Note 3 . The Complete Ease simulation software was used to fit the measured values of the real and imaginary parts of the dielectric tensor to psi and delta of the different samples. Spectroscopic reflection and transmission measurements were carried out on a Olympus BX51 microscope with × 20 magnification and detected with an Ocean Optics QE 65,000 spectrometer. 3D-nanowire-like nanostructures in PS and Bi 2 Te 3 For the fabrication of the 3D nanowire-like periodic nanostructures made of PS, the 3D AAO was submerged into styrene (Aldrich Ltd.) for 1 h to induce the infiltration of the monomer into the tubular cavity. Then the styrene was polymerized using AIBN (Aldrich Ltd.) as initiator under N 2 atmosphere. In the case of Bi 2 Te 3 , it was electrodeposited into the 3D AAO template for 8 h pulsing 0.1 s at 20 mV and 0.1 s at J =0 mA cm −2 versus Ag/AgCl [34] . A potentiostat-galvanostat (Eco Chemie, Model AUT302.0) and a three-electrode cell were used for electrodeposition. 3D nanocomposites of 3D AAO and functional polymers To fabricate the composite materials, 3D AAOs were infiltrated with 4 g l −1 chloroform solutions of PCDTBT, fluorene, thiophene and benzothiazole copolymer, poly(3-ethyl acetate thiophene-2,5-diyl), poly(phenylene vinylene) and 5 wt% solution of poly(vinylidene flouride-co-trifluoroethylene) in dimethylformamide. How to cite this article : Martín, J. et al. Ordered three-dimensional interconnected nanoarchitectures in anodic porous alumina. Nat. Commun. 5:5130 doi: 10.1038/ncomms6130 (2014).